Flexible and twistable non-volatile memory cell array with all-organic one diode–one resistor architecture Flexible organic memory devices are one of the integral components for future flexible organic electronics. However, high-density all-organic memory cell arrays on malleable substrates without cross-talk have not been demonstrated because of difficulties in their fabrication and relatively poor performances to date. Here we demonstrate the first flexible all-organic 64-bit memory cell array possessing one diode–one resistor architectures. Our all-organic one diode–one resistor cell exhibits excellent rewritable switching characteristics, even during and after harsh physical stresses. The write-read-erase-read output sequence of the cells perfectly correspond to the external pulse signal regardless of substrate deformation. The one diode–one resistor cell array is clearly addressed at the specified cells and encoded letters based on the standard ASCII character code. Our study on integrated organic memory cell arrays suggests that the all-organic one diode–one resistor cell architecture is suitable for high-density flexible organic memory applications in the future. Organic-based electronic devices have been intensively investigated in recent decades because of their potential advantages over conventional inorganic electronics, such as their light weight, flexibility, roll-to-roll printing compatibility and the ease of tailoring their optoelectronic properties [1] , [2] , [3] , [4] , [5] , [6] , [7] , [8] , [9] , [10] . Recently, various publications have described highly efficient organic solar cells and organic transistors with integrated logic circuits and remarkably low operating voltages [11] , [12] , [13] , [14] , [15] . Organic memory devices have also been explored for data storage applications [2] , [3] , [4] , [16] , [17] . Most research on organic memory devices has focused on the development of new materials or the demonstration of their operation in a simple device structure. For commercial applications, more research is required to scale down the dimensions of the cell while using advanced cell architectures, effectively pattern the active materials to isolate neighbouring cells in a cross-bar array and fabricate memory cells on flexible substrates [2] , [18] , [19] , [20] . With regard to minimization of array dimensions, it is well known that a cross-bar array has the highest cell density in a two-dimensional planar device structure (4 F 2 where F represents the minimum feature size) [21] . However, in the cross-bar array structure, unintended current leakage paths can lead to the misreading of memory states within the cells (commonly called ‘cross-talk’ between neighbouring cells), and it must be eliminated to achieve precise memory switching operation. In order to solve this cross-talk problem, another functional device should be combined with the memory device. One transistor–one resistor (1T–1R) and one diode–one resistor (1D–1R) can potentially alleviate this cross-talk problem [20] , [22] . However, these approaches have been based on a hybrid (organic/inorganic) device structure and could not be printed on flexible substrates or take full advantage of the solution processibility of organic materials. Recently, 1D–1R memory devices with exclusively organic active materials (excluding electrodes) and organic bistable rectifying diodes have been reported [23] , [24] . However, they were not demonstrated on flexible substrates with a high density of cells, nor did they exhibit essential memory characteristics, such as retention, endurance, in situ pulse response and exhaustive testing, during and after physical stresses. To realize these benchmarks, the active organic materials should be processible at low temperatures to facilitate device fabrication on flexible substrates. In addition, to enhance memory characteristics, the subsequent thin films must be patternable on a desired area and resistant to spin coating of successive layers from organic solutions without eroding. These are essential requisites for not only the integration of organic non-volatile memory arrays on flexible substrates but also the fabrication of organic non-volatile memory cells with advanced architectures and highly reliable performance. Furthermore, both pulse response and precise addressing tests should be carried out on single cells and the entire cell array to examine accurate operation and practical use in organic electronic applications. In this study, we fabricate ultraviolet-patterned and vertically stacked 64-bit 1D–1R memory cell arrays using poly(3-hexylthiophene) (P3HT) diodes and a mixture of polystyrene (PS) and 6-phenyl-C 61 butyric acid methyl ester (PCBM) for the memory components on polyethylene naphthalate (PEN) flexible substrates at low temperature. The memory and diode devices were patterned using a photoactive crosslinker (bis-perfluorobenzoazide: Bis-FB-N 3 ) to covalently link the PS and P3HT side chains via nitrene-based N-H insertion reactions, which confers solvent resistance to the active layers [25] . Each individual memory and diode device in the integrated memory cell work without malfunction. The 64-bit 1D–1R memory cell arrays also show stable memory characteristics ( I ON / I OFF ratio ~10 3 ) and reliable retention times (10 4 s) and endurance cycles (10 2 cycles) after substrate deformation, which is likely to happen during practical use. In addition, the issue of undesired cross-talk between neighbouring cells is solved by integrating the organic diodes directly on top of the organic memory cells. No cross-talk is observed after various mechanical deformations of the flexible substrate. Even during bending deformation, the 1D–1R memory cells are found to respond perfectly to input voltage pulses. Moreover, specific letters are encoded with the 64-bit memory cell array based on the standard ASCII character code. 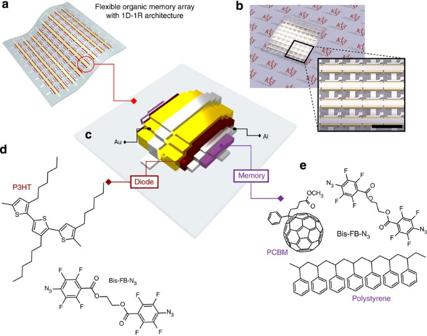Figure 1: Flexible all-organic 1D–1R cell. (a) Illustration of as-fabricated 1D–1R organic resistive memory cell array on a flexible PEN substrate and (b) optical image. Scale bar, 5 mm. (c) Schematic of unit cell of 1D–1R cell (Al/PS:PCBM/Al/P3HT/Au/Al). (d) Chemical structure of P3HT and Bis-FB-N3for ultraviolet patternable diode layer. (e) Chemical structure of PS, PCBM and Bis-FB-N3for ultraviolet patterable memory layer. Flexible all-organic 1D–1R cell array Figure 1 depicts the structure and materials employed in the flexible memory cell array integrated in a vertically stacked 64-bit 1D–1R architecture developed in this work. Typically, multi-layer organic frameworks experience poor performance or device failure because of erosion during layer-by-layer processing. To avoid this erosion, Bis-FB-N 3 was used to crosslink the alkyl chains in P3HT thin films via light-catalysed N-H insertion reactions [25] . The Bis-FB-N 3 acts as a negative photoresistor responding to 254 nm ultraviolet light and allows patterning of common alkylated organic materials [23] , [25] . Crosslinking with Bis-FB-N 3 imbues the organic layer with a robust resistance against common organic solvents used for spin coating. In addition, Bis-FB-N 3 is one of the few crosslinkers that are compatible with temperature-sensitive plastic substrates. In our previous work, an ultraviolet patternable polyimide (PI) and PCBM blending solution was chosen as a memory component on a rigid substrate, because the PI has good chemical robustness after imidization [23] . Unfortunately, the imidization temperature of PI is known as over 250 °C and this issue allows limited use of PI on plastic substrate. Most existing crosslinkers require high temperatures to initiate the crosslinking reaction, which destroys plastic substrates. However, the use of a light-activated crosslinker enables low-temperature processing conditions (~90 °C), which plastic substrates can withstand [26] , [27] . This approach might be a more efficient way to process multiple organic-soluble layers than use of orthogonal solvents [28] . Figure 1a,b shows an illustration and optical image of an as-fabricated all-organic 64-bit 1D–1R memory cell array on a PEN substrate. The entire integrated structure of the 1D–1R cell is (bottom) PEN/Al/PS:PCBM/Al/P3HT/Au/Al (top), as shown in Fig. 1c . A P3HT/Bis-FB-N 3 solution was chosen as the diode material ( Fig. 1d ), and a PS/PCBM/Bis-FB-N 3 mixture was used for the unipolar memory component ( Fig. 1e ). Figure 1: Flexible all-organic 1D–1R cell. ( a ) Illustration of as-fabricated 1D–1R organic resistive memory cell array on a flexible PEN substrate and ( b ) optical image. Scale bar, 5 mm. ( c ) Schematic of unit cell of 1D–1R cell (Al/PS:PCBM/Al/P3HT/Au/Al). ( d ) Chemical structure of P3HT and Bis-FB-N 3 for ultraviolet patternable diode layer. ( e ) Chemical structure of PS, PCBM and Bis-FB-N 3 for ultraviolet patterable memory layer. Full size image To determine whether each device element worked properly in the vertically stacked architecture, an electrical characterization was performed as shown in Fig. 2 . 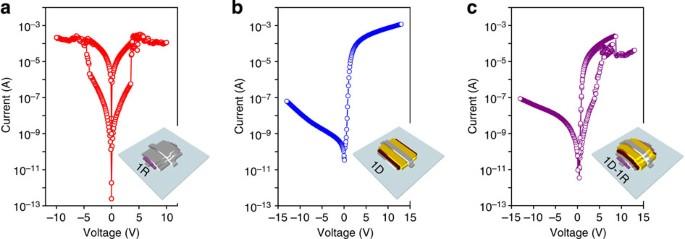Figure 2: Memory characteristics of 1R and 1D and 1D–1R cell. I–Vcurve of (a) memory-only cell (1R cell in patterned 1R cell array), (b) diode-only cell (1D cell in patterned 1D cell array) and (c) vertically integrated 1D–1R cell in patterned 1D–1R cell array. Figure 2a shows a current–voltage ( I – V ) graph of a ultraviolet-patterned memory cell (Al/PS:PCBM/Al). It was turned on (set) at 3.5 V and completely turned off (reset) at 10 V, exhibiting typical unipolar switching behaviour. The memory switching seems to result from the polarization of the PCBM clusters and generation of a strong electric field between adjacent clusters [29] . The I ON / I OFF ratio of the devices was greater than 10 3 (at 1.5 V). Figure 2b depicts a rectification curve of an integrated P3HT schottky diode (Al/P3HT/Au). It exhibits the expected rectification behaviour with a high-rectification ratio of 10 5 . Figure 2: Memory characteristics of 1R and 1D and 1D–1R cell. I – V curve of ( a ) memory-only cell (1R cell in patterned 1R cell array), ( b ) diode-only cell (1D cell in patterned 1D cell array) and ( c ) vertically integrated 1D–1R cell in patterned 1D–1R cell array. Full size image This P3HT diode prevents cross-talk between cells caused by parasitic current paths in a cross-bar array architecture [2] , [18] . To eliminate the cross-talk problems associated with memory-only (1R) cell arrays, a P3HT diode is vertically integrated onto each memory cell by spin coating a P3HT film over the memory cells, then using a shadow mask to ultraviolet pattern the diodes directly on top of each memory cell, as shown in the inset of Fig. 2c . Unlike the I – V curve of 1R cells ( Fig. 2a ), the memory cells with a vertically integrated organic diode (1D–1R cell) retained their inherent memory characteristics in the forward bias regime because of the ohmic contact between the Au electrode (work function: 5.1 eV) and P3HT diode (HOMO: 4.9 eV). On the other hand, the memory cells showed limited current flow in the reverse bias regime because of the Schottky barrier between the Al electrode (work function: 4.1 eV) and P3HT diode (HOMO: 4.9 eV). For this reason, the Al middle electrodes were inserted between the memory and diode. The all-organic flexible 1D–1R memory cell was set around 4 V and completely reset at 13 V. The relatively high operation voltage compared with the memory-only cell might be due to series resistance between the memory and diode components. The electrical properties of the flexible 1D–1R memory cells were characterized using Keithley 4200-SCS and Hewlett and Packard 4145B semiconductor parameter analyser in a N 2 -filled glove box. Various mechanical distortions In order to investigate how the 64-bit all-organic flexible 1D–1R memory cell array behaved under various physical stresses, we first performed electrical characterization of the flexible 1D–1R cells while they were bent ( Fig. 3a,b ). The PEN substrate (30.3 × 30.3 mm 2 ) holding the 1D–1R cell was bent from flat to a radius of curvature ( r ) of ~13 mm (strain of 0.48%) using a home-made holder made from vernier calipers. The detailed information on bending method and estimation of strain are shown in Supplementary Fig. S1 (refs 30 , 31 , 32 ). As shown as Fig. 3a , the memory device was completely functional, even after bending (strain of 0.48%). 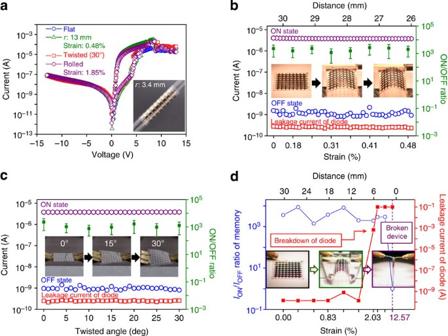Figure 3: Memory characteristics of flexible 1D–1R cell. (a)I–Vcurve of 1D–1R cell before, after bending, twisted and rolled. (b)I–Vcharacteristic of 1D–1R cell under gradual bending and statisticalION/IOFFratio distribution of 1D–1R cell under gradual bending. (c)I–Vcharacteristic of 1D–1R cell and statisticalION/IOFFratio distribution during gradual twisting. (d)ION/IOFFratio and leakage current of diode until device malfunction. Figure 3: Memory characteristics of flexible 1D–1R cell. ( a ) I – V curve of 1D–1R cell before, after bending, twisted and rolled. ( b ) I – V characteristic of 1D–1R cell under gradual bending and statistical I ON / I OFF ratio distribution of 1D–1R cell under gradual bending. ( c ) I – V characteristic of 1D–1R cell and statistical I ON / I OFF ratio distribution during gradual twisting. ( d ) I ON / I OFF ratio and leakage current of diode until device malfunction. Full size image For more realistic applications of our all-organic flexible 1D–1R cell, we did in situ current measurements at the ON, OFF and leakage currents of the organic diode while the flexible substrate was gradually bent. After being turned ON, the ON state current value was monitored during gradual bending. Interestingly, it did not show large current variation regardless of bending as shown in Fig. 3b (purple hexagons). Similarly, the OFF state current was monitored after the device was turned off under identical bending conditions. The devices displayed consistent OFF current values, as shown in Fig. 3b (blue circles). The 1D–1R cell was measured in the reverse bias regime of the P3HT diode under the same bending conditions and it retained consistent leakage current values ( Fig. 3b , red squares). The ON and OFF currents were read at 1.5 V (forward bias regime of 1D–1R cell) and the leakage current was read at −1.5 V (reverse bias regime of the 1D–1R cell). Regardless of the magnitude or change of the bending radius (increasing strain), the 1D–1R cell retained function of the memory and diode components (resistive change or rectification). To examine the operational uniformity of the device, I ON / I OFF ratios were statistically analysed on 40 working cells under gradual bending conditions. The devices showed high I ON / I OFF ratio (~10 3 ) from flat to bending with strain of 0.48% ( Fig. 3b ) and high I ON / I OFF ratios (~10 3 ) during 10 4 times bending cycles ( Supplementary Fig. S2a ). One bending cycle means the device was bent to strain of 0.48% and subsequently relaxed to flat. There were negligible I ON / I OFF ratio fluctuations, showing a consistent I ON / I OFF ratio of ~10 3 . The retention test was also performed on cells with increased bending cycle times. The retention time of the memory devices was stable and reliable, even up to 10 4 bending cycles over 10 4 s ( Supplementary Fig. S2b ). In addition to the bending test, the memory cell array was distorted in other ways. As shown in Fig. 3a,c , we twisted the flexible 1D–1R memory cell array using home-made equipment and measured twisting angles with a protractor ( Supplementary Fig. S3 ). Interestingly, there was not a significant change in I – V curves before and after stressing the substrates at the maximum twist angle (30°). The 1D–1R cell current values were measured in the forward (ON, OFF) and reverse (leakage current of diode) regimes to evaluate whether the flexible 1D–1R devices could withstand gradual twisting stresses. They showed consistent current (ON, OFF and diode leakage) as shown in Fig. 3c , regardless of the twisting angle. The I ON / I OFF ratios were statistically analysed on 40 working cells under gradual twisting. They kept their I ON / I OFF ratios of ~10 3 from flat to 30° ( Fig. 3c ). The 1D–1R cell showed stable retention characteristics for more than 10 4 s, even while the device was twisted by 30° ( Supplementary Fig. S2c ). Envisioning an extreme stress condition, the cell array was rolled on a glass pipet with a radius of 3.4 mm (strain of 1.85%) as shown in the inset of Fig. 3a . Despite the small bending radius, the 1D–1R cell worked properly and showed stable retention characteristics over 10 4 s ( Supplementary Fig. S2c ). The detailed descriptions on roll method are illustrated in Supplementary Fig. S4 . These results indicate that the all-organic flexible 1D–1R cells have robust operation and reliable electrical properties even under harsh substrate physical deformation. Furthermore, we bent the device more severely to figure out the 1D–1R cell failure during bending condition. The diode (1D) showed malfunction of rectification (10 −4 A) in negative polarity at strain of 2.03% ( r ~3.1 mm) as shown in Fig. 3d . In contrast, the memory (1R) was normally operating showing ~10 3 of I ON / I OFF ratio. In order to figure out the malfunction of memory, the device was more bent. The memory was working normally showing ~10 3 of I ON / I OFF ratio until strain of 6.28% ( r ~1 mm). However, the memory was broken at strain of 12.57% ( r ~0.5 mm) as shown in Fig. 3d . The detailed information on malfunction of 1D and 1R is explained in Supplementary Figs S5 and S6 . The strain value of each radius of curvature is listed in Supplementary Table S1 . The pulse-response signal of 1R and 1D–1R cells was tested to determine the fidelity of the write-read-erase-read (WRER) sequence. There have been negligible reports about this measurement on integrated organic memory devices with advanced architectures and under physical stresses. 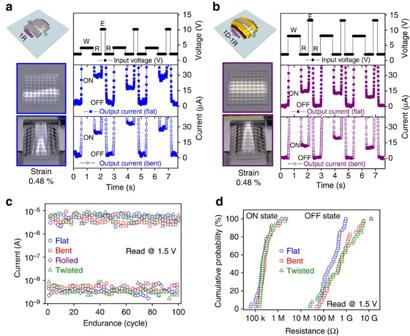Figure 4: Pulse response and reliability test of flexible 1D–1R cells. Write-read-erase-read (WRER) cycle test of (a) 1R cell and (b) 1D–1R cell. The graph in the top shows input voltage pulse of (a) 1R cell and (b) 1D–1R cell. The graph in the middle indicates output current response before bending of (a) 1R cell and (b) 1D–1R cell. The graph in the bottom exhibits output current response after bending (a) 1R cell and (b) 1D–1R cell. (c) Endurance cycles and (d) cumulative probability on various substrate distortion of 1D–1R cell. Figure 4a,b shows the results of the WRER test on 1R and 1D–1R cells. The top graph of Fig. 4a shows the input voltage pulse signal applied to the 1R cell. The cell was subjected to a 900-ms write pulse at 4 V and a subsequent 300-ms erase pulse at 10 V and was read at a voltage of 2 V. The middle and bottom graphs of Fig. 4a show the output current response of the 1R cell before and after bending with strain of 0.48% ( r ~13 mm). The memory cell was completely responsive at input signals at current transitions (ON, OFF). The top of Fig. 4b shows the input voltage of the 1D–1R memory cell. A 900-ms write pulse at 8 V, a 300-ms erase pulse at 13 V and a read voltage at 2 V were used for the response test. Although the operation voltage was increased because of the diode element, the integrated cell exhibited great behaviour, showing outstanding switching current values (ON, OFF state) before and after bending with strain of 0.48% ( r ~13 mm), as shown in the middle and bottom of Fig. 4b . Endurance cycles and cumulative probability of the flexible 1D–1R device were evaluated when the device was flat, bent, rolled and twisted. As shown in Fig. 4c , the flexible 1D–1R device showed reliable functions without current overlap for both ON and OFF currents even up to 10 2 cycles. In order to check device operational uniformity, the resistance of ON and OFF current were statistically analysed on 40 working cells under various substrate deformation (bent, twisted) as shown in Fig. 4d . The ON and OFF resistances were perfectly segregated, and the ON current, in particular, showed narrow distribution. The WRER cycles were measured with a two-channel pulse generator (Agillent Technology, 81104A) and a four-channel oscilloscope (Tektronix, DPO 4104B). Figure 4: Pulse response and reliability test of flexible 1D–1R cells. Write-read-erase-read (WRER) cycle test of ( a ) 1R cell and ( b ) 1D–1R cell. The graph in the top shows input voltage pulse of ( a ) 1R cell and ( b ) 1D–1R cell. The graph in the middle indicates output current response before bending of ( a ) 1R cell and ( b ) 1D–1R cell. The graph in the bottom exhibits output current response after bending ( a ) 1R cell and ( b ) 1D–1R cell. ( c ) Endurance cycles and ( d ) cumulative probability on various substrate distortion of 1D–1R cell. Full size image Addressing test In order to figure out the effect of vertically integrated diode, a current addressing test was executed for 1R devices (memory only), using 1D–1R devices for comparison. As shown in the inset of Fig. 5a , an OFF current (that is, the ‘0’ state) was applied to one cell of the 1R device. Subsequently, an ON current (that is, the ‘1’ state) was applied to three adjacent cells. Then, the current was read at each of the four cells at 1.5 V. In the 1R device, the ON and OFF currents were not correctly read because of cross-talk between the neighbouring cells ( Fig. 5b ). Despite programming one cell to an OFF current (~10 −8 A), all the cells displayed ON currents (~10 −5 A), as shown in the left histogram of Fig. 5c . The same experiment was carried out on the 1D–1R device as shown as Fig. 5d . Unlike the 1R device, the 1D–1R device shows precise addressing ( Fig. 5e ). In the 1D–1R device, the current state of the OFF cell was read correctly. Owing to the vertically integrated diode, the reverse current path (bottom to top electrodes) was blocked because of the Schottky barrier but the forward current path (top to bottom electrodes) was open because of ohmic contact. Thus, the information in the OFF state can be perfectly read as shown in the right histogram of Fig. 5c . Verifying the accurate addressing in the 64-bit 1D–1R memory cell array, we wrote ‘KIST’ as shown in Fig. 5f . The letters of ‘KIST’ were programmed based on the ON (1) and OFF (0) currents by the standard ASCII character code in 3 × 3 cells (for each letter) among the 8 × 8 cells array 1D–1R device. 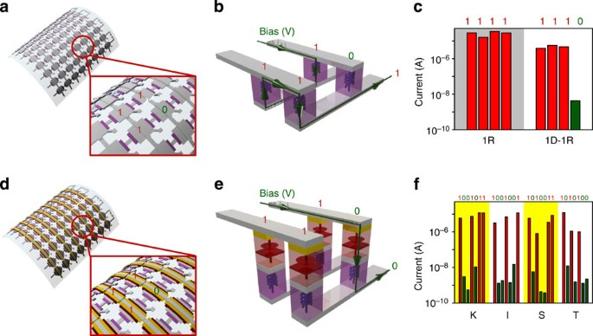Figure 5: Addressing test of 1R and 1D–1R cells. (a) Programmed current states of 1R cells. (b) Current path without stacked diode (1R cells). (c) Histogram of current states during the reading process of 1R cells and 1D–1R cells. (d) Programmed current states of 1D–1R cells. (e) Current path with stacked diode (1D–1R cells). (f) The output currents histogram exhibiting the letter ‘KIST’ by the standard ASCII characters within the 8 × 8 1D–1R cells. Figure 5: Addressing test of 1R and 1D–1R cells. ( a ) Programmed current states of 1R cells. ( b ) Current path without stacked diode (1R cells). ( c ) Histogram of current states during the reading process of 1R cells and 1D–1R cells. ( d ) Programmed current states of 1D–1R cells. ( e ) Current path with stacked diode (1D–1R cells). ( f ) The output currents histogram exhibiting the letter ‘KIST’ by the standard ASCII characters within the 8 × 8 1D–1R cells. Full size image We fabricate a 64-bit all-organic flexible memory cell array in a 1D–1R architecture with photopatternable organic memory (PS:PCBM) and diode (P3HT) systems. Light-catalysed crosslinking enables low-temperature materials processing, which thereby allows device fabrication on a flexible PEN substrate, resulting in the first fully flexible memory device. These 1D–1R cells showed good electronic behaviour and rewritable switching, even during and after harsh physical stresses. They retain their respective current values (ON, OFF and leakage current of the diode) during gradual substrate deformation without sacrificing their individual electrical properties. The 1D–1R cells show stable retention characteristics over 10 4 s even while undergoing substrate distortion up to 10 4 bending cycles. An in situ measurement of the response signal via the external pulse signal with WRER sequences reveals that our 1D–1R cell array is a candidate for practical use in high-density all-organic flexible memory applications. Furthermore, the all-organic flexible 1D–1R cell array successfully avoids cross-talk problems and can write specific letters based on standard ASCII character code, illustrating promising operational performance for practical flexible organic memory applications. Also, the 1D–1R cells show reliable reproducibility and uniformity regardless of mechanical device deformation. Our research represents one of the initial key studies describing the fabrication and characterization of integrated flexible organic electronics exploiting sophisticated architectures. Material preparations In order to prepare the memory cell active material, PS (7 mg) and PCBM (1 mg) were dissolved into chlorobenzene (1 ml) with Bis-FB-N 3 (5 mg) to make the ultraviolet patternable solution. For preparation of the organic diode solution, P3HT (55 mg) was dissolved in chlorobenzene (1 ml) with Bis-FB-N 3 (5 mg). Fabrication of flexible 1D–1R cell array A 125-μm-thick PEN substrate (30.3 × 30.3 mm 2 ) was prepared for the flexible 1D–1R memory device and cleaned by acetone and isopropyl alcohol. The 70-nm thick Al bottom electrodes were deposited using a shadow mask by a thermal evaporator with a deposition rate of 5 Å s −1 at a pressure of ~10 −7 torr. The Al bottom electrodes deposited on the PEN substrate were exposed to ultraviolet-ozone to increase film uniformity [33] . The prepared memory solution was filtered through a 0.45-μm polytetrafluoroethylene filter and spin coated onto the substrate at 500 r.p.m. for 5 s and then at 1,000 r.p.m. for 60 s. After spin coating, the substrate was exposed to ultraviolet (254 nm) light using a shadow mask for 5 min to initiate the crosslinking reaction, then rinsed with chlorobenzene at 4,000 r.p.m. for 60 s. The patterned device was annealed at 90 °C for 10 min in a N 2 filled glove box. As the top electrodes of the memory cells and the bottom electrodes of diode cells, 70 nm thick Al middle electrodes were deposited by thermal evaporator using a shadow mask. The prepared diode solution was spin coated at 1,500 r.p.m. for 60 s and then exposed to ultraviolet (254 nm) light using a shadow mask for 5 min to initiate crosslinking then rinsed with chlorobenzene at 4,000 r.p.m. for 60 s. As the top electrodes for the diode, Au electrodes (100 nm) were deposited by a thermal evaporator using a shadow mask. For the arrayed 1D–1R device, the Al top electrodes were deposited by thermal evaporator using a shadow mask. The detailed fabrication process information is described in the Supplementary Fig. S7 . The thickness of the memory layer was ~70 nm and the diode layer was ~300 nm ( Supplementary Fig. S8 ). How to cite this article: Ji, Y. et al. Flexible and twistable non-volatile memory cell array with all-organic one diode–one resistor architecture. Nat. Commun. 4:2707 doi: 10.1038/ncomms3707 (2013).